High rates of anaerobic methane oxidation in freshwater wetlands reduce potential atmospheric methane emissions The role of anaerobic oxidation of methane (AOM) in wetlands, the largest natural source of atmospheric methane, is poorly constrained. Here we report rates of microbially mediated AOM (average rate=20 nmol cm −3 per day) in three freshwater wetlands that span multiple biogeographical provinces. The observed AOM rates rival those in marine environments. Most AOM activity may have been coupled to sulphate reduction, but other electron acceptors remain feasible. Lipid biomarkers typically associated with anaerobic methane-oxidizing archaea were more enriched in 13 C than those characteristic of marine systems, potentially due to distinct microbial metabolic pathways or dilution with heterotrophic isotope signals. On the basis of this extensive data set, AOM in freshwater wetlands may consume 200 Tg methane per year, reducing their potential methane emissions by over 50%. These findings challenge precepts surrounding wetland carbon cycling and demonstrate the environmental relevance of an anaerobic methane sink in ecosystems traditionally considered strong methane sources. Freshwater wetlands (FWW) are characterized by high rates of methanogenesis, and although they occupy a small fraction of the Earth’s surface, they represent one of the largest natural sources of methane to the atmosphere [1] . Few studies have examined anaerobic oxidation of methane (AOM) in FWW [2] , [3] , [4] , [5] and AOM was largely regarded as inconsequential in these environments until recently. Instead, aerobic methane oxidation was assumed to be the dominant mode of methane consumption in FWW [6] . The reasoning for this assumption is simple: sulphate was long considered the sole oxidant for methane [7] in anoxic environments and sulphate is scarce in freshwater. In marine environments, where sulphate is available in much higher concentrations, AOM exerts a strong control over methane fluxes from the seabed [8] . Yet, despite low sulphate concentrations, FWW support a dynamic sulphur cycle and high rates of sulphate reduction [9] (SR) are maintained by rapid recycling of reduced sulphur species [10] . Moreover, studies of freshwater AOM have indicated several electron acceptors for methane oxidation, including sulphate [11] , nitrate/nitrite [5] , [12] , [13] , [14] , [15] , iron [16] and manganese [17] . Geochemical profiles [4] , [18] , [19] , stable isotope geochemistry [16] , [18] , [19] , potential methane oxidation assays [2] , [4] , [5] , [20] and long-term enrichments [4] have provided tantalizing evidence of AOM in FWW, but environmentally relevant, in vitro , rate measurements are rare [9] . This study provides the first constraints on both the magnitude and extent of AOM in FWW, a critical first step to understanding the role of this process in freshwater environments. 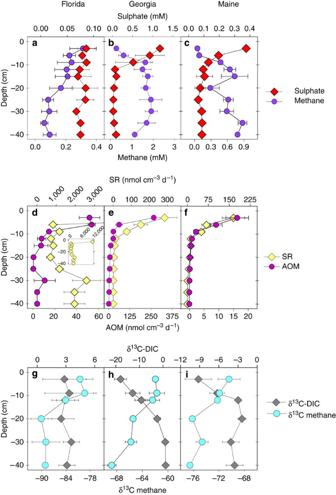Figure 1: Geochemistry and microbial activity with depth in freshwater wetland sediment and peat. Data are a mean (n=3)±s.e.m. (a–c) Profiles of methane (purple circles) and sulphate (red diamonds) in Florida, Georgia and Maine (left to right). (d–f) Rates of AOM (fuschia circles) and SR (yellow diamonds). The inset ondshows the full scale for SR in the same units as the primary panel. (g–i) Stable carbon isotopic signatures (δ13C) of DIC (grey diamonds) and of methane (sky blue circles). Data from Florida collected in January 2010, from Georgia in August 2008 and from Maine in March 2009. AOM, anaerobic oxidation of methane; DIC, dissolved inorganic carbon; SR, sulphate reduction. We investigated AOM in three FWW across distinct biogeographical provinces: the freshwater peat soils of the Florida Everglades, a coastal organic-rich wetland in Acadia National Park, Maine, and a tidal FWW in coastal Georgia ( Table 1 ). All three sites were sampled in at least two different seasons. This suite of sampling sites captured a range of in situ conditions (average temperature, climate conditions, organic matter content and so on) to illustrate the broad relevance of AOM in FWW. We employed in vitro radiotracer assays to quantify rates of AOM and SR, and quantified porewater chemistry and stable carbon isotope geochemistry, including that of microbial lipid biomarkers, to evaluate the magnitude of AOM, its role in wetland carbon cycling, and the microbial community potentially involved in AOM. Table 1 Geochemical characterization and microbial activities in freshwater wetland sediment and peat. Full size table Rates of AOM Considerable reservoirs of porewater methane were present in these FWW pore fluids, all of which supported high rates of biological methane production [21] ( Table 1 ). The anoxic, permanently water-saturated surface soils (see Methods) exhibited the highest rates of AOM ( Fig. 1 ), although AOM was detected at all depths examined (down to 40 cm). Maximal rates (>265±9 nmol cm −3 per day) of AOM were observed in Georgia ( Fig. 1 ), with lower, more similar AOM rates observed in Maine and Florida (maxima of 16±4 and 54±3 nmol cm −3 per day, respectively). Substantial AOM rates were sustained across a range of in situ temperatures and seasons ( Supplementary Table 1 ). Surprisingly, AOM rates in the sediments and peat are comparable to those reported for deep-sea methane seeps [22] and coastal marine sediments [7] . These in vitro rate measurements provide some of the first concrete evidence of AOM in FWW [9] ( Fig. 1 ). Figure 1: Geochemistry and microbial activity with depth in freshwater wetland sediment and peat. Data are a mean ( n =3)±s.e.m. ( a–c ) Profiles of methane (purple circles) and sulphate (red diamonds) in Florida, Georgia and Maine (left to right). ( d–f ) Rates of AOM (fuschia circles) and SR (yellow diamonds). The inset on d shows the full scale for SR in the same units as the primary panel. ( g–i ) Stable carbon isotopic signatures (δ 13 C) of DIC (grey diamonds) and of methane (sky blue circles). Data from Florida collected in January 2010, from Georgia in August 2008 and from Maine in March 2009. AOM, anaerobic oxidation of methane; DIC, dissolved inorganic carbon; SR, sulphate reduction. Full size image Sulphate reduction and sulphur cycling The wide range of SR rates measured during this study fell within the range of values reported for FWW [23] . The combination of high SR rates and low sulphate concentrations (78–247 μM on average; Fig. 1 ) led to short turnover times for sulphate (2–5 days), and thus required rapid reoxidation of reduced sulphur species, as observed in other wetlands [10] . This reoxidation may have occurred in the uppermost mm of peat/sediment [24] , which were exposed to oxygenated bottom waters and to the atmosphere by diurnal tides at the site in Georgia, or via anaerobic oxidation coupled to nitrate [25] , oxidized trace metals [26] , humic substances [27] , or nanowires [28] , any of which could serve as electron sinks. 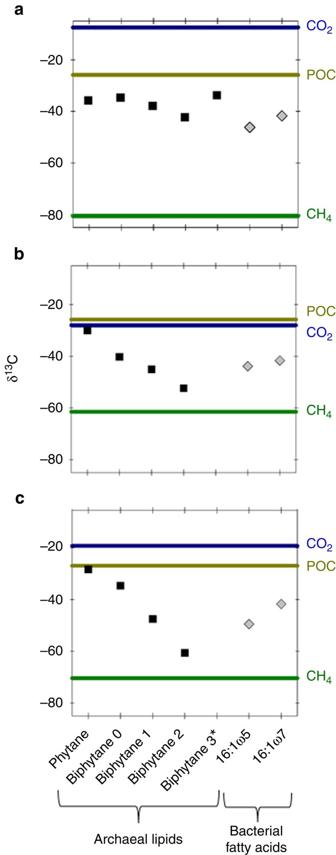Figure 2: Stable isotopic composition of microbial lipids in freshwater wetlands. Displayed is the range of the stable carbon isotopic signature (δ13C) of selected archaeal (black squares) and bacterial (grey diamonds) intact-derived core lipids compared against the δ13C of methane (CH4; green line), particulate organic carbon (POC; brown line), and dissolved carbon dioxide (CO2; blue line) in the zone of maximum activity of anaerobic oxidation of methane (0–3 cm). Isotope values are an average based onn=1–2 measurements for lipids andn=3 for geochemical species which were derived from triplicate cores. (a) Data from Florida in January 2010. (b) Data from Georgia in August 2008. (c) Data from Maine in March 2009. Archaeal core lipids were analysed as phytanes derived from archaeol and hydroxyarchaeol and biphytanes with 0–3 rings derived from glyceroldialkylglycercol-tetraethers. The most depleted bacterial core lipids detected at all three sites (16:1ω5 and 16:1ω7) are also shown. *The concentration of biphytane 3 was not sufficient to generate a robust isotopic signal in Georgia (b) or Maine (c). Dissolved hydrogen sulphide (HS − ) concentrations were undetectable in Georgia and low (0.3–7.8 μM) in Maine and Florida ( Table 1 ), suggesting that HS − is either quickly reoxidized or scavenged via precipitation of reduced metal, likely iron [29] sulphides, as Fe oxides are abundant in these wetlands, especially in Georgia ( Supplementary Table 2 ). This precipitation, in addition to rapid oxidation of free sulphides by poorly crystalline iron and manganese [30] , likely account for the low to undetectable HS − concentrations despite high SR rates. Possible electron acceptors for AOM In marine habitats the majority of AOM is mediated by methanotrophic archaea (ANME) that oxidize methane with sulphur in association with sulphate-reducing bacteria [7] , [31] , [32] . In contrast, a dominant electron acceptor for freshwater AOM has not been identified. Experimental evidence suggest sulphate is not the sole electron acceptor for AOM in freshwater sediments and peat [2] , [9] , [15] , [20] , and AOM in low-sulphate environments has been linked to the reduction of nitrate, nitrite, iron and manganese [4] , [5] , [12] , [13] , [16] , [33] . The geochemical and rate profiles in the wetlands studied here support a linkage between SR and AOM. The upper sediment/peat horizons at all three sites supported maximal activities of AOM and SR ( Fig. 1 ). Rates of AOM were significantly correlated with rates of SR at all sites ( r =0.78; P <0.01) as well as with sulphate concentrations in Georgia and Maine ( r =0.9; P <0.01). In most samples, SR rates were sufficient to support AOM; SR in excess of AOM was likely fuelled through hydrogenotrophic or heterotrophic mechanisms [34] . Previous studies compared the magnitude of AOM and SR rates to determine how closely the two processes are coupled [22] , [35] . At depth (>9 cm) in Georgia sediments, AOM rates were significantly ( P <0.05) higher than SR. Thus, while AOM in Maine and Florida may be coupled to SR, at least some fraction of AOM activity in Georgia must be supported by alternative electron acceptor(s). Such alternative electron acceptors (for example, nitrate, nitrite, iron oxides or manganese oxides) were readily available in these sediments ( Table 1 ; Supplementary Table 2 ) and may support AOM in FWW [5] , [9] , [13] . The production of reduced iron at depth in Georgia ( Supplementary Fig. 1e ) could suggest Fe-oxide-fuelled AOM rates in excess of SR, as previously documented in long-term incubations with these sediments [9] . Profiles of reduced iron concentrations were highly correlated with AOM in Florida ( r =0.80; P <0.05), which could reflect either rapid reoxidation of AOM-derived HS − by iron oxides or direct coupling of AOM and iron reduction ( Supplementary Figs 1a and 2d ). However, in long-term incubations with sediment from Georgia the addition of sulphate elicited higher rates of potential AOM than did the addition of iron, manganese or nitrate [9] and maximal AOM rates were observed in slurries without any added electron acceptors. This and other evidence of AOM in FWW without anthropogenically-enhanced nitrogen levels indicate an as-yet-unidentified electron acceptor [2] , [20] . While nitrite has been shown to support AOM in some nitrogen enriched wetlands [5] , [36] , the evidence for nitrate-dependent anaerobic methane oxidation (n-damo) in this study is weak. AOM was not significantly correlated with nitrite concentrations in Florida or Georgia. In Maine, the correlation between nitrite and AOM ( r =0.83; P <0.05) was weaker than the correlation of AOM and sulphate ( r =0.98; P <0.01) or SR ( r =0.97; P <0.01). Humic substances, which are plentiful in these organic-rich wetlands, are a possible candidate [3] . Humic acids can serve as electron acceptors/shuttles in other anaerobic metabolisms and the addition of humic acids lowered methane emissions from a peatland, possibly through stimulation of AOM [37] . Their importance has only yet been implied where the addition of inorganic electron acceptors has dampened AOM rates [9] , [20] . The results of this study do not necessarily advance this theory, as rates of AOM were not correlated with concentrations of dissolved organic carbon or with soil organic content. Still, a connection between AOM and humic acid reduction remains a tantalizing possibility. Possible impacts on methane emissions Direct consumption of methane via AOM-limited methane emissions from these FWW. AOM rates in excess of methane production from hydrogen and acetate highlights the effectiveness of AOM in reducing methane emissions within the sedimentary horizon examined ( Supplementary Fig. 2 ). Additional methane to support the measured oxidation rates may have been produced from alternative substrates [38] and/or supplied via vertical advection from depths >40 cm or lateral advection [21] in the tidally-influenced sites (Georgia and Florida). In addition to AOM, competitive limitation of methanogenesis by other terminal metabolisms may also contribute to reductions in methane fluxes in these FWW. The ratio of SR to methanogenesis ( Table 1 ) and the suppression of methanogenesis in the zones of maximum SR activity in Florida and Georgia ( Supplementary Fig. 2 ) suggest that SR limited methane production in horizons where sulphate was present, further limiting methane emissions through thermodynamic energetic restrictions on methane production [39] . Isotopic evidence of AOM In addition to quantifying rates of AOM and SR, we evaluated the impact of AOM on microbial carbon flow in these wetlands by measuring the stable carbon isotopic composition (δ 13 C) of methane, dissolved inorganic carbon (DIC) and intact microbial lipids. Biological consumption results in 13 C enrichment of residual methane through the preferential consumption of isotopically light methane [40] . The zone of maximum AOM activity (0–3 cm) corresponded to the lowest δ 13 C-DIC values and the highest δ 13 C-CH 4 , a clear geochemical signature of AOM ( Fig. 1 ) that corroborated the radiotracer results. This pronounced porewater isotopic signal, along with AOM measurements made during other seasons ( Supplementary Table 1 ), indicate sustained AOM activity at these sites. In the marine environment, lipid biomarkers are robust indicators of metabolic coupling between methane-oxidizing archaea and their sulphate-reducing bacterial partners: both groups of microorganisms exhibit lipids that are highly depleted in 13 C relative to methane, indicating assimilation of methane-derived carbon through AOM [7] , [41] . However, results from freshwaters are inconsistent: some evidence of extreme depletion of 13 C in microbial lipids [14] has been noted while others report little to no depletion in lipid isotopic signatures [11] , [16] . Despite the clear importance of AOM in these wetlands, as established by the δ 13 C profiles of DIC and methane and the measured rates of AOM ( Fig. 1 ), a classic methanotrophic signal was absent in the isotopic signature of microbial lipids ( Fig. 2 ). Figure 2: Stable isotopic composition of microbial lipids in freshwater wetlands. Displayed is the range of the stable carbon isotopic signature (δ 13 C) of selected archaeal (black squares) and bacterial (grey diamonds) intact-derived core lipids compared against the δ 13 C of methane (CH 4 ; green line), particulate organic carbon (POC; brown line), and dissolved carbon dioxide (CO 2 ; blue line) in the zone of maximum activity of anaerobic oxidation of methane (0–3 cm). Isotope values are an average based on n =1–2 measurements for lipids and n =3 for geochemical species which were derived from triplicate cores. ( a ) Data from Florida in January 2010. ( b ) Data from Georgia in August 2008. ( c ) Data from Maine in March 2009. Archaeal core lipids were analysed as phytanes derived from archaeol and hydroxyarchaeol and biphytanes with 0–3 rings derived from glyceroldialkylglycercol-tetraethers. The most depleted bacterial core lipids detected at all three sites (16:1ω5 and 16:1ω7) are also shown. *The concentration of biphytane 3 was not sufficient to generate a robust isotopic signal in Georgia ( b ) or Maine ( c ). Full size image Generally, the greatest 13 C depletions were observed in lipids within the surface sediment/peat horizons, where maximal AOM activities were observed ( Fig. 2 ; for example Fig. 1 ). The most diagnostic lipids were archaeal mono- and bi-cyclic biphytanes ( Fig. 2 ; Supplementary Table 3 ), as reported previously for deep anoxic waters in the Black Sea [42] . These compounds are derived from polar glycerol dialkyl glycerol tetraethers with one to three cyclopentane moieties and are particularly abundant in marine sediments hosting AOM communities [43] , while they are not observed in known (cultured isolates) methanogens [44] . The δ 13 C values of these lipids (−60.6 to −36.8‰) are still within the range considered diagnostic of AOM in marine settings [7] , [42] ; however, they are relatively heavy given that they are enriched in 13 C relative to porewater methane at all the three sites ( Fig. 2 ). The isotopic enrichment of archaeal lipids relative to methane is best explained by additional biological sources of these compounds, for example, from heterotrophic archaea [45] or autotropic archaea such as ammonium-oxidizing thaumarcharchaea [46] . Alternatively, the incorporation of DIC rather than methane into methane-oxidizing archaeal lipids [47] could explain the observed 13 C-enriched values. Notably, the archaeal biphytanes are 13 C-depleted relative to CO 2 by −42 to −17‰, consistent with a predominant origin from autotrophic, methane-oxidizing archaea [47] . The most strongly 13 C-depleted bacterial lipids detected in all three FWW (minimum value −49.5‰) were C 16:1ω5 and C 16:1ω7 ( Fig. 2 ; Supplementary Table 3 ). These lipids are typically associated with sulphate-reducing bacteria at methane-rich seeps where their 13 C-depletion signals an association with sulphate-reducing bacteria (SRB) involved in sulphate-dependent AOM [41] . Their lower δ 13 C values compared with the other fatty acids in these FWW suggest a methanotrophic influence. 10-Methyl-hexadecanoic acid, a characteristic lipid for ‘ Methylomirabilis oxyfera ’, a freshwater bacterium capable of oxidizing methane with nitrite [33] , was either not detected at these sites or found in rather low abundance (<1.5% of all fatty acids; data not shown). This proposed biomarker for n-damo [48] was not sufficiently depleted in 13 C to unambiguously support a relationship with AOM ( Supplementary Table 3 ); a conclusive relationship of this biomarker to AOM is complicated by the evidence for chemoorganoautotrophy of M. oxyfera [49] , in analogy to some ANME archaea [47] , and additional sources of this biomarker such as sulphate-reducing [50] and anammox bacteria [51] . The other proposed diagnostic lipid for M. oxyfera , 10-methyl-hexadec-7-enoic acid [48] , was not detected in any sample. The anaerobic oxidation of methane serves as a major methane sink in marine environments and effectively limits fluxes of this greenhouse gas from the oceans to the atmosphere [8] . While the body of evidence for AOM in FWW is growing, direct rate measurements are rare [9] . This is the first comprehensive study of methanotrophy in FWW to document actual (versus potential) rates of AOM. We measured activity down to a depth of 40 cm (the deepest horizon sampled) in 270 samples. Rates were sustained over a range of in situ temperatures ( Table 1 and Supplementary Table 1 ), suggesting this process is widespread in FWW systems throughout the year. Strikingly, the FWW rates are comparable in magnitude with those documented in marine systems [35] , [52] . AOM rates were similar to or exceeded rates of methane production from acetate and hydrogen (the two major methanogenic substrates [53] ) within the depth range assayed ( Table 1 ). These results, along with previous experimental results [9] , [20] , highlight the potentially large role AOM plays in wetland methane cycling. Further attention to this topic is justified in order to better constrain the global methane budget and the role of FWW in past and present climate dynamics. In marine settings, AOM is widespread and believed to be coupled largely to SR [7] , [32] , [35] . In comparison, there is no convergence on the dominant mechanism for AOM in freshwater environments [3] , [5] , [9] , [16] , [17] . The available empirical evidence is contradictory. Many experiments with FWW soils have shown that the addition of sulphate, iron, nitrate or manganese does not enhance AOM activity relative to a control [2] , [5] , [9] , [20] . Recent studies have found high abundances of Ca. M. oxyfera and affiliated members of this phylum in FWW [4] , [5] . However, to date evidence for n-damo originated in freshwater environments with high nitrogen loading and most published rates are from long-term enrichments [5] , [36] , [54] , [55] . The conditions of such experiments do not fully mimic in situ conditions, as they are often conducted after prolonged preincubation phases, with additions of methane and electron acceptors, and with slurried material. It is therefore difficult to determine how these results translate to natural settings. Thus, while there is a growing body of literature supporting an important role of n-damo in methane biogeochemistry of FWW and rice paddies, there are several lines of evidence that suggest n-damo was not the dominant process of methane oxidation in the FWW examined here. For one, the wetlands of this study are fairly pristine with very low nitrite concentrations and maximum nitrate concentrations of ∼ 80 μM ( Supplementary Fig. 1 ). The porewater profiles of methane and nitrate were distinct and uncorrelated. Furthermore, peak AOM activity occurred in the surface sediments of these wetlands, while n-damo has been detected in deeper depths where nutrient-laden porewaters dominate (at least 20 cm and typically between 50 and 80 cm depth) [36] , [54] . The lipid biomarker data also does not support a strong influence of n-damo. And finally, long-term incubations with slurried sediment from Georgia and amended with nitrate resulted in lower rates of AOM than compared with additions of sulphate, iron or the control [9] . The concomitant rate maxima for SR and AOM in the same depth horizons, along with significant correlations between the rates of these two processes ( r =0.85, P <0.01) indicate that sulphate may support the bulk of the AOM measured in this study. However, alternative electron acceptors remain feasible. Sulphate-independent AOM is clearly indicated at some depth horizons in Georgia where rates of AOM exceeded rates of SR. On the basis of previous, long-term incubations with this soil [9] , we posit that iron and/or humic substances may play a role. Experimental additions of humic substances may prove useful in future investigations. Wetlands are highly dynamic settings that receive large inputs of organic matter and support diverse metabolic activities. While we detected some imprint of AOM on the isotopic composition of microbial lipids, representative ‘superlight’ lipids that typify deep-sea hotspots of AOM were absent in these three FWW ( Supplementary Table 3 ). The breakdown of organic matter from a myriad of sources (for example, grasses, trees and other allochthonous sources) likely leads to an admixture of isotopic signals in the pools of carbon dioxide, acetate and other low-molecular weight substrates in these wetlands. This is in contradiction to marine methane seeps where methane is the dominant organic carbon source, thus generating a more uniform signal. A methanotrophic signal in microbial lipids may also have been obscured by autotrophic and heterotrophic activities (for example, nitrate, sulphate, iron, and manganese reduction and methanogenesis) which utilize carbon substrates more enriched in 13 C than methane and produce less 13 C-depleted lipids [56] . Alternatively, freshwater anaerobic methanotrophs may be metabolically distinct from their deep-sea counterparts, which may exhibit metabolic plasticity depending on environmental conditions [57] . Elucidating the microorganism(s) involved in AOM in these systems is not possible based on biomarker and δ 13 C values alone. Some have argued the extreme isotopic depletions in archaeal lipids attributed to AOM in vent and seep communities may be entirely due to autotrophic methanogenesis [58] . Recent isotope-based inquiries, however, have demonstrated that microorganisms involved in AOM assimilate carbon dioxide [47] , [57] in addition to methane [57] . Phylogenetic analyses indicate variable AOM pathways likely occur, possibly within a single group of archaea in response to environmental factors [57] . The failure to detect ‘superlight’ archaeal lipids does not exclude methanotrophic or methanogenic activity, both of which are important in these wetlands [9] . Furthermore, microorganisms mediating AOM in FWW may be utilizing unrecognized metabolic pathways, thus producing lipids with distinct isotopic compositions. Using an average areal AOM rate within the top 40 cm from the three sites across multiple years and seasons ( Table 1 ; Supplementary Table 1 ) and an estimated global wetland area [59] of 5.69 × 10 12 m 2 , AOM is estimated to consume around 200 Tg methane per year, or nearly as much methane as is emitted from global FWW on an annual basis [1] . While this estimate is derived from only three wetlands, these sites represent three distinct biogeographical provinces that were sampled multiple times across different seasons. Limiting the comparison to temperate wetlands [60] (0.6–1.1 × 10 12 m 2 ), AOM may consume between 20 and 40 Tg methane per year, or 1–30 times the estimated annual methane flux from these environments [60] , [61] . In a direct comparison, atmospheric methane flux measurements [21] were roughly twice the magnitude of areally-integrated AOM rates in Georgia in August 2008. Clearly, AOM serves as a crucial gatekeeper that modulates methane emissions from both freshwater and marine environments [8] . Coastal wetlands are vulnerable to sea-level rise and increased sulphate availability via saltwater intrusion is likely to decrease methane production and dampen methane emissions from these ecosystems [39] . As sea levels rise, increased sulphate loading may further reduce methane fluxes by limiting methane production and stimulating AOM. As FWW ecosystems are responsible for a major portion of global emissions, a better constraint of methane cycling in wetlands is paramount to understanding past and future global methane budgets and the role of FWW in the global methane cycle. Site descriptions Sediment/peat cores were collected from wetlands within three distinct biogeographical provinces: Caribbean (Florida), Carolinian (temperate; Georgia) and Acadian (cold-temperate; Maine). The study site in Florida is located within the Florida Coastal Everglades LTER at Shark River Slough (25° 49′ N, 80° 41′ W). The peat was ∼ 1 m thick, lay atop a bed of marl, and contained an average of 81% organic material with an average carbon to nitrogen ratio (C:N; by weight) of 15. The marsh at Shark River Slough was dominated by Cladium jamaicense interspersed with Eleocharis and Panicum , though no living macrophytes were present in the peat sampled. While the Everglades are typified by a distinct wet (May to November) and dry (December to April) season, this site remains inundated throughout the year. Anoxic peat samples were collected from Florida in September 2009 and January 2010. The site in coastal Georgia was located along Hammersmith Creek (31° 20′ N, 81° 28′ W), a tidal, freshwater creek that feeds into the Altamaha River. Adjacent to the creek bank is a marsh dominated by Zizaniopsis miliacea . The sediments in Georgia are fine-grained silt and clays with an average organic content of 17% and an average C:N of 12. Maximum water depths at high tide range from about 0.5 (neap) to 2 m (spring) and oxygen is consumed within the top 3 mm of sediment (personal observations). Anoxic sediments were collected in January, April and August 2008 and in February and November 2009. The study site in Maine was located on the north side of Mount Desert Island in Acadia National Park. Samples were collected in Aunt Betsey’s Brook (44° 24′ N 68° 18′ W), a freshwater creek which runs into the Fresh Meadow and eventually into Thomas Bay. The site was visited in late winter (March 2009) and again in late summer (August 2009). Anoxic sediments were collected from the unvegetated creek bed, which is permanently inundated with freshwaters. A 3–10 cm layer of ice, which had formed over the brook in the winter of 2009, was manually removed from the sampling area before cores were taken. The surrounding marsh is dominated by Spartina pectinata, Scirpus acutus and Typha . The organic-rich soil in Maine contained an average organic matter content of 33% with an average C:N of 17. Sample collection and geochemical analysis At least six sediment or peat cores were collected within a 2–3 m 2 area of unvegetated peat or sediment. This number afforded a minimum of three replicate cores for all analyses. Cores were processed under a stream of argon either in the field or within 24 h on return to the laboratory, where they were sectioned at 3–5 cm intervals to a depth of 40 cm and processed for geochemical analyses and rate assays. Triplicate cores were processed for geochemical analyses. For methane analysis, a 6 cm 3 peat/sediment sample was taken from each sub-core with a cutoff plastic syringe. These plugs were preserved in a helium-purged serum vial containing 3 ml 2 N sodium hydroxide (final pH<13) and sealed with a blue, butyl-rubber stopper and a crimp seal. Samples were stored at room temperature until analysis on a Shimadzu GC-2014 gas chromatograph (GC) equipped a flame-ionization detector (FID) and a Carbosphere column. A 1 cm 3 sample was collected into tared glass vials for porosity and loss-on-ignition determination [35] . The porewaters in each sediment/peat horizon were extracted into an argon-purged syringe using a mechanical squeezer and argon-purged squeezer cups [35] . A portion of this extracted porewater was preserved for DIC analysis by injecting 5 ml of porewater into a helium-purged gas vial containing 200 μL of 6 N hydrochloric acid and fitted with a blue, butyl-rubber stopper and crimp seal. The liberated carbon dioxide in the headspace was analysed using a GC-FID outfitted with a methanizer after the vial was shaken vigorously. A 10 ml aliquot of the porewater was 0.2 μm filtered (to halt microbial activity) and stored frozen for acetate, nitrite and nitrate analysis. Another 10 ml aliquot was 0.2 μm filtered and preserved for sulphate, iron (II) and manganese (II) by addition of 100 μl 16 M trace-metal grade nitric acid. A 2 ml sample for HS − was preserved by adding 200 μl 20% zinc acetate to 2 ml of porewater. Concentrations of nitrate, nitrite, sulphate, dissolved iron (II), manganese (II) and HS − were determined using standard, previously published protocols (as described by Segarra et al. [9] ). Concentrations of total solid-phase iron and manganese were determined by subjecting the peat/sediment to a hot 6 N hydrochloric acid extraction [62] followed by analysis on a flame atomic absorption spectrophotometer. Concentrations of acetate were determined using high-performance liquid chromatography [63] (HPLC). Microbial activity assays Three additional cores were processed for microbial rate measurements of AOM, methanogenesis and SR. Using the same depth horizons as those sub-sampled for geochemistry, subcores of peat/sediment for each rate measurement from each horizon were collected in to a cut-end glass Hungate tubes and sealed with a moveable black butyl-rubber stopper at one end and a black butyl-rubber septa and open-hole screw cap at the other. These airtight tubes were stored at in situ temperature for 24 h before beginning radiotracer incubations. This acclimation period served to allow the microbial population to recover from any possible transport and handling disturbance as well as to scavenge any available oxygen. Microbial activities were calculated as volume-specific (nmol cm −3 per day) and as depth-integrated (mmol m −2 per day) rates (via trapezoidal integration of the volume-specific rates in the top 40 cm of sediment). All rates were porosity corrected when appropriate. Base-killed controls (pH>13) were incubated in parallel for each process within each depth interval so that live samples could be corrected for this ‘background’ activity. To assure robust rate data, we evaluated the linearity of the targeted process over time in radiotracer assays (data not shown). Short incubation times in this linear period were used to minimize tracer turnover. Methods for determining rates of AOM were published previously [9] . Briefly, ∼ 11.7 kBq of 14 CH 4 tracer was injected and live samples were incubated for 24 h alongside killed controls for each depth interval. The tracer added <6 nmol methane which increased the extant methane concentration by 3% or less. To terminate activity and preserve produced 14 CO 2 as carbonate, 5 ml of 2 N sodium hydroxide was injected through the rubber septum. The product ( 14 CO 2 ) was recovered by acid digestion and the activity of both the product and tracer were determined via liquid scintillation counting [64] . The recovery rate of labelled 14 CO 2 was >97% and limit of detection for AOM assays was 0.1 nmol cm −3 per day. Rates of hydrogenotrophic methanogenesis ( 14 CH 4 from H 14 CO 3 − ) and acetoclastic methanogenesis ( 14 CH 4 from 2- 14 CH 3 COO − ) were performed, processed and calculated using previously published methods [52] . The recovery rate of labelled methane was >95%. The average activity of the H 14 CO 3 − tracer was 380 kBq. The average activity of the added 2- 14 CH 3 COO − was 160 kBq with a specific activity of 1.7–2.2 GBq mmol −1 . Methods for the SR rate measurements were identical to those of Segarra et al. [9] . The limit of detection for SR was 2.0 × 10 −3 nmol cm −3 per day. Lipid extraction For lipid analysis, between 3 and 33 g of frozen sediment or peat were homogenized by hand with a solvent-cleaned Teflon spatula. Larger amounts of material were extracted from greater depths than the surface due to the generally lower lipid yields with depth. Lipids were extracted using a modified Bligh-Dyer extraction protocol [65] , [66] . The total lipid extract was separated into a polar, intact lipid fraction and a non-polar fraction using preparative HPLC with a fraction collector, similar to the methods in Kellermann et al. [67] except that only two fractions were collected: polar and apolar. Proper separation of these two fractions was validated by liquid chromatography–mass spectrometry (see protocol below). Stable isotope analyses Stable carbon isotope ( 13 C) measurements were performed on porewater methane and DIC, particulate organic carbon, and microbial core lipids and reported in δ 13 C notation (‰) relative to the Vienna Peedee Belemnite Standard. Stable carbon isotope compositions of methane (δ 13 C-CH 4 ) and δ 13 C-DIC were analysed at the Center for Applied Isotope Studies at the University of Georgia with a Thermo Scientific Delta V Plus isotope ratio mass spectrometer (IRMS). Before isotopic analysis, methane and carbon dioxide were separated with an Agilent HP 6,890 GC on a Carboxen 1,006 Plot column with a helium carrier at 100 °C interfaced with a Thermo Scientific Delta V Plus GC combustion module. Measurements were performed in duplicate on each triplicate sub-sample. The δ 13 C of carbon dioxide was calculated from δ 13 C-DIC with the in situ temperature according to Mook et al. [68] For isotopic analysis of particulate organic carbon, replicate ( n =3) sediment horizons were dried, homogenized and combined before removal of inorganic carbon via fuming with hydrochloric acid and analysis with an elemental analyser coupled to an IRMS. The stable carbon isotopic composition of apolar derivatives of intact polar lipids were analysed with a ThermoFinnigan Trace GC coupled to a ThermoFinnigan Delta-plus XP IRMS via GC-combustion interface III to a HP Series GC [69] . The precision of replicate analysis ( n =2) of selected samples was better than 1‰. Before compound-specific δ 13 C analysis, apolar derivatives of the intact polar lipids were produced using standard protocols; the methods used for each lipid class are briefly described below. Polar lipid fatty acids (PLFAs) and polar neutral lipids were obtained via saponfication of an aliquot of the polar total lipid extract using methods described previously [41] , [69] . The PLFA and neutral products were stored in n -hexane at −20 °C until derivatization and analysis by GC-FID. The PLFA products were derivatized with methanolic BF 3 and analysed as fatty acid methyl esters with GC-FID [70] . The neutral lipid fractions (containing alcohols and ether lipids, such as monoalkyl glycerol ethers and dialkyl glycerol ethers) were derivatized with bis-(trimethylsilyl)trifluoroacetamide at 70 °C for 1 h. Apolar derivatives of ether-bound intact polar archaeal lipids were obtained using a protocol for ether cleavage involving BBr 3 and subsequent reduction of the resulting alkylbromides [69] , [70] . The ether-based products (phytanes and biphytanes) were stored in n-hexane at −20 °C until analysis on the GC-IRMS without derivatization. How to cite this article: Segarra, K. E. A. et al. High rates of anaerobic methane oxidation in freshwater wetlands reduce potential atmospheric methane emissions. Nat. Commun. 6:7477 doi: 10.1038/ncomms8477 (2015).